Low energy carbon capture via electrochemically induced pH swing with electrochemical rebalancing We demonstrate a carbon capture system based on pH swing cycles driven through proton-coupled electron transfer of sodium (3,3′-(phenazine-2,3-diylbis(oxy))bis(propane-1-sulfonate)) (DSPZ) molecules. Electrochemical reduction of DSPZ causes an increase of hydroxide concentration, which absorbs CO 2 ; subsequent electrochemical oxidation of the reduced DSPZ consumes the hydroxide, causing CO 2 outgassing. The measured electrical work of separating CO 2 from a binary mixture with N 2 , at CO 2 inlet partial pressures ranging from 0.1 to 0.5 bar, and releasing to a pure CO 2 exit stream at 1.0 bar, was measured for electrical current densities of 20–150 mA cm −2 . The work for separating CO 2 from a 0.1 bar inlet and concentrating into a 1 bar exit is 61.3 kJ mol CO2 −1 at a current density of 20 mA cm −2 . Depending on the initial composition of the electrolyte, the molar cycle work for capture from 0.4 mbar extrapolates to 121–237 kJ mol CO2 −1 at 20 mA cm −2 . We also introduce an electrochemical rebalancing method that extends cell lifetime by recovering the initial electrolyte composition after it is perturbed by side reactions. We discuss the implications of these results for future low-energy electrochemical carbon capture devices. Accumulating CO 2 emissions from anthropogenic activities constitute the major cause of global climate change [1] , [2] . While efforts are being made in switching from fossil fuel-based energy to virtually emissions-free sources such as nuclear, solar, wind and geothermal, fossil fuel combustion will remain an important component of the world economy for a long time [3] . Consequently, carbon removal—whether captured from a point source [2] , [4] , [5] , [6] , [7] , [8] such as a combustion power plant or directly from the air (a.k.a. direct air capture, DAC) or the ocean [2] , [9] , [10] , [11] , [12] , [13] —in order to reduce atmospheric CO 2 concentrations, is gaining increasing attention. Numerous methods for point source capture and DAC have been developed. Among the most studied is wet amine scrubbing for point source capture [4] , [5] , [6] and strongly alkaline (pH > 14) solution for DAC [2] , [9] , both of which rely on a large temperature-swing cycle to regenerate sorbents. Although sorbent composition has been optimized to lower the energy cost for both strategies, the thermal energy requirement for heating is still ~100 kJ mol CO2 −1 for point source capture [6] , [14] , [15] and >150 kJ mol CO2 −1 for DAC [10] , [16] . In addition, sorbent volatility, toxicity, and corrosivity cause environmental concerns [2] . Methods that remove CO 2 from the ocean, which allow it to absorb more CO 2 , have also been studied, but the high water-handling requirement is a challenge [12] , [13] . Electrochemically mediated separation technologies constitute an increasingly attractive alternative to traditional temperature-swing or pressure-swing methods because of the rapidly decreasing cost of intermittent renewable electricity and the mild operating conditions of ambient temperature and pressure [7] , [8] , [13] , [17] , [18] , [19] , [20] . However, most existing methods operate at low current density (<5 mA cm −2 ) because of large overpotentials and the corresponding energetic cost at higher current density, implying a high capital cost of electrochemical hardware. Recently, our group proposed and demonstrated a pH swing cycle for CO 2 separation electrochemically driven through proton-coupled electron transfer (PCET) of redox active organic molecules (“Q”) [18] . In this scheme, proton-coupled electrochemical reduction of these molecules (Q + 2H 2 O + 2 e − → QH 2 + 2OH − ) raises the electrolyte pH and total alkalinity (TA), leading to CO 2 capture from point source or air and conversion to dissolved inorganic carbon (DIC); subsequent electrochemical oxidation of the reduced molecules (QH 2 + 2OH − → Q + 2H 2 O + 2 e − ) acidifies the electrolyte and lowers TA, resulting in the conversion of DIC to CO 2 gas and its release. Here, we report a proof-of-concept point source (10%) CO 2 separation system that uses a sodium (3,3′-(phenazine-2,3-diylbis(oxy))bis(propane-1-sulfonate)), i.e., DSPZ (Fig. 1a ), based electrochemical pH-swing cell with an energy cost of only 61.3 kJ mol CO2 −1 at 20 mA cm −2 . Through analyzing the cycle work obtained under systematically varied inlet partial pressure and current density, we estimate that the cost for capturing from a 0.4 mbar CO 2 inlet using this system extrapolates to 121– 237 kJ mol CO2 −1 at 20 mA cm −2 , and that it can be further lowered if a higher concentration of DSPZ, or other PCET-active molecules, is used. Recognizing the sensitivity of the reduced form of DSPZ, i.e., DSPZH 2 , to chemical oxidation by atmospheric or dissolved O 2 , we introduce and demonstrate an electrochemical rebalancing method that expels oxygen from solution and restores the initial composition of the electrolytes. Fig. 1: Scheme of the pH swing carbon capture flow system. a Schematic of the reversible PCET (proton-coupled electron transfer) reaction underwent by DSPZ (sodium (3,3′-(phenazine-2,3-diylbis(oxy))bis(propane-1-sulfonate))) in an aqueous solution. b Schematic of the Fe(CN) 6 (posolyte) | DSPZ (negolyte) flow cell and full system. Blue arrows indicate gas flow direction. Adapted from ref. [18] . c Process flow. TA is total alkalinity and DIC is dissolved inorganic carbon. The solid arrows refer to desired reactions in a complete carbon capture/release cycle. The carbonate formation and decomposition reactions are neglected for simplicity. The dashed arrow on the right side refers to the side reaction caused by oxygen and the dashed arrow on the left refers to reactions in the electrochemical rebalancing step. Full size image 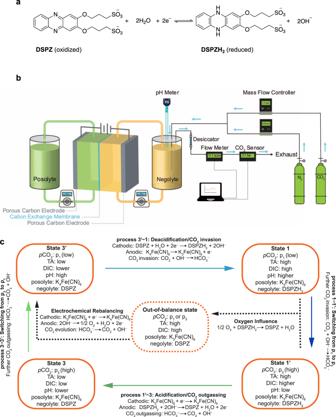Fig. 1: Scheme of the pH swing carbon capture flow system. aSchematic of the reversible PCET (proton-coupled electron transfer) reaction underwent by DSPZ (sodium (3,3′-(phenazine-2,3-diylbis(oxy))bis(propane-1-sulfonate))) in an aqueous solution.bSchematic of the Fe(CN)6(posolyte) | DSPZ (negolyte) flow cell and full system. Blue arrows indicate gas flow direction. Adapted from ref.18.cProcess flow. TA is total alkalinity and DIC is dissolved inorganic carbon. The solid arrows refer to desired reactions in a complete carbon capture/release cycle. The carbonate formation and decomposition reactions are neglected for simplicity. The dashed arrow on the right side refers to the side reaction caused by oxygen and the dashed arrow on the left refers to reactions in the electrochemical rebalancing step. Device setup and process flow Figure 1b shows the schematic of the Fe(CN) 6 |DSPZ carbon capture flow cell and the hardware for providing the gas mixture and analyzing the exhaust. The upstream gas composition in the negolyte headspace was controlled by CO 2 and N 2 mass flow controllers (MFCs). Downstream of the negolyte reservoir, the gas was dried with a desiccator and the total gas flow rate and CO 2 partial pressure were measured using a digital flow meter and a CO 2 sensor, respectively. A pH probe immersed in the negolyte solution reported the temporal evolution of its pH, which enabled the tracking of total alkalinity (TA) and dissolved inorganic carbon (DIC) in real time. Figure 1c illustrates the electrolyte composition in the four states of the pH swing carbon capture cycle and the processes connecting the states. We denote the CO 2 partial pressure during the CO 2 capture process as the inlet pressure or p 1 , and that during the CO 2 outgassing process as the exit pressure or p 3 , which is always set to 1 bar (100% CO 2 ) in this study. Similarly, the subscripts following TA or DIC refer to the TA and DIC of the corresponding states. The naming convention for the states is adopted from previous work [18] , where the equilibrium and constraints governing pH, TA, DIC, and p CO 2 are explained in detail. The four colored arrows in Fig. 1c refer to the four processes in the carbon capture cycle. The four sequential processes are as follows: 3′ i →1: two-stage deacidification+CO 2 invasion (inlet). In this process, DSPZ is electrochemically reduced to DSPZH 2 , and hydroxide is produced, which reacts with CO 2 to form carbonate/bicarbonate. 1→1′: change of the headspace atmosphere from inlet to exit pressure, i.e., switching from p 1 to p 3 . 1′→3: two-stage acidification+CO 2 outgassing (exit). In this process DSPZH 2 is electrochemically oxidized to DSPZ and hydroxide is consumed, which in turn leads to carbonate/bicarbonate decomposition and CO 2 evolution. 3→3′ f : change of the headspace atmosphere from exit to inlet pressure, i.e., switching from p 3 to p 1 . The change in TA and DIC in these processes are denoted with ΔTA a→b and ΔDIC a→b , respectively, where the subscript refers to process “a→b”, and a and b are any pairs of states. An example cycle is described quantitatively in the next section. As DSPZH 2 is reversibly chemically oxidized by atmospheric O 2 to DSPZ (right dashed arrow in Fig. 1c ), the posolyte supplies extra charge to electrochemically reduce the extra oxidized DSPZ; this is reflected in the low Coulombic efficiency of the cell and an accumulation of TA and DIC in the negolyte. This process also transforms more of the posolyte to its oxidized form, i.e., [K + ] 4 [Fe II (CN) 6 ] 4− → [K + ] 3 [Fe III (CN) 6 ] 3− + K + + e − , than at a similar point in the previous deacidification-acidification cycle. During cell operation reduction on one side must be accompanied by oxidation on the other side but, as the available fraction of reduced species on the posolyte side, i.e., [K + ] 4 [Fe II (CN) 6 ] 4− , decreases, the cell can access less and less of its theoretical capacity during its oxidation-reduction oscillations; this is reflected in the decaying capacity of the cell. Eventually, both sides become 100% oxidized and cell operation ceases. Our remedy for such situations is the electrochemical rebalancing method (left dashed arrow in Fig. 1c ) explained later in the text. One carbon capture cycle with p 1 = 0.1 bar and p 3 = 1 bar at 40 mA cm −2 In previous work we demonstrated a series of non-concentrating cycles, in which both exit and inlet p CO 2 were 0.47 bar, utilizing a DSPZ-based flow cell at 40−150 mA cm −2 [18] . In the present work, we show the use of this setup for CO 2 separation from low partial pressure in a mixture with nitrogen and release into a pure CO 2 exit stream at 1.0 bar. 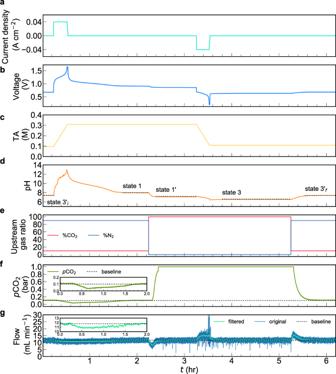Fig. 2: A CO2concentrating cycle with inlet pressurep1= 0.1 bar and exit pressurep3= 1 bar using a DSPZ-based flow cell at 40 mA cm−2. Electrolytes comprised 10 mL 0.11 M DSPZ in 1 M KCl (negolyte, capacity limiting) and 35 mL 0.1 M K4Fe(CN)6and 0.04 M K3Fe(CN)6in 1 M KCl (posolyte, non-capacity limiting).aCurrent density.bVoltage.cTotal alkalinity.dpH of the negolyte. States 3′i, 1, 1′, 3 and 3′frepresent pH values before deacidification under 0.1 barpCO2, after deacidification+absorption under 0.1 barpCO2, after changingpCO2from 0.1 bar to 1 bar, after acidification+desorption under 1 bar and after changingpCO2from 1 bar to 0.1 bar, respectively. The detailed composition of these states is elaborated in Table1.eN2and CO2percentage in the upstream source gas, controlled by mass flow controllers.fDownstream CO2partial pressure. The baseline indicatespCO2= 0.1 bar. Inset: Zoomed-in view of downstream CO2partial pressure in between 0 <t< 2 h, where CO2capture takes place.gDownstream total gas flow rate; the baseline is 11.8 mL min−1. Inset: Zoomed-in view of downstream gas flow rate (filtered) in between 0 <t< 2 h, where CO2capture takes place. Figure 2 demonstrates one such cycle with p CO 2 = 1.0 and 0.1 bar at the exit and inlet, respectively. Beginning at state 3′ i , the upstream CO 2 partial pressure was set to 0.1 bar, which is close to its value in the flue gas from coal fired power plants [7] . We define t as the time elapsed. As deacidification began (Fig. 2a, b , t = 0.2 h), the TA went up at a linear rate because only K + ions crossed the cation exchange membrane (CEM) when a constant 40 mA cm −2 current density was applied (Fig. 2c ) [18] . 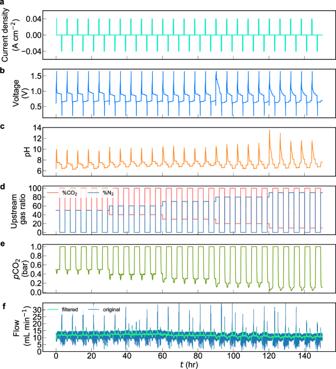Fig. 3: Twenty five CO2concentrating cycles with 0.5, 0.4, 0.3, 0.2, and 0.1 bar inlet pCO2 and 1 bar exit pCO2 at 40 mA cm−2. Same cell and negolyte as in Fig.2were employed. aCurrent density.bVoltage.cpH of the negolyte.dN2and CO2percentage in the upstream source gas, controlled by mass flow controllers; total pressure 1.0 bar.eDownstream CO2partial pressure.fDownstream total gas flow rate. As a result of the PCET reactions during the reduction of DSPZ, the negolyte pH (Fig. 2d ) increased from near neutral to ~13.5 at the end of the deacidification process, indicated by the steep increase of voltage until reaching the preset voltage cutoff of 1.65 V (Fig. 2b , t = 0.6 h). CO 2 invasion began when deacidification began but continued beyond the end of deacidification: invasion lasted until t = 1.8 h, as indicated by the p CO 2 signal returning to the 0.1 bar baseline, because of the limited reaction rate between dilute OH − and CO 2 . The deviation in the gas flow rate (Fig. 2g ) from the baseline starting at t = 0.2 h and returning at 1.8 h also documents the complete capture process. As CO 2 reacted with hydroxide and water to form CO 3 2− and HCO 3 − , the pH (Fig. 2d ) dropped from ~13.5 at t = 0.5 h to 8.1 at 1.8 h and then plateaued, once again indicating the completion of the capture process. The absorbed volume of CO 2 is 47 mL (Eq. ( 1 ) in “Methods”). Assuming T = 293 K, p = 1 bar, and ideal gas behavior, this absorption causes a change in DIC of 0.20 M (2.0 mmol CO 2 in 10 mL negolyte volume). We denote this change as ΔDIC flow,3 ′ i→1 , where the subscript “ flow ” indicates that the value is measured by the downstream flowmeter and CO 2 sensor and “ 3 ′ i → 1” indicates that this value corresponds to the change in process 3′ i →1 (Table 1 ). The same naming convention is used for both ΔTA and ΔDIC throughout the rest of this text. 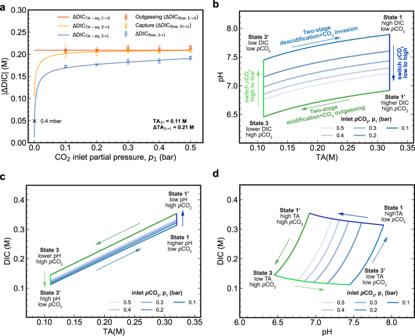Fig. 4: Summary of the experimental concentrating cycles with different inletpCO2in Fig.3and the TA (total alkalinity)/pH/DIC (dissolved inorganic carbon) relations of the ideal cycles with corresponding experimental conditions. aΔDICflowextracted from Fig.3e, f(colored “x” markers) and calculated ΔDICTA−eqgiven TA3′i= 0.11 M and ΔTA3→1= 0.21 M (lines). The black “x” marker refers to the result that ΔDIC for the ideal cycle equals 0.049 M whenpCO2= 0.4 mbar. The error bars refer to the standard deviation.bpHvs. TA in the ideal cycles, assuming TA3′i= 0.11 M, ΔTA3→1= 0.21 M and gas-solution equilibrium.p1in the legends representspCO2during the two-stage deacidification+CO2invasion process. The arrows indicate the direction of the processes in the experiments.cDICvs. TA in the ideal cycles.dDICvs. pH in the ideal cycles. Unlike the flowmeter and CO 2 sensor, which quantify ΔDIC, the pH probe, in addition to providing a measured value (pH meas ), provides a direct measurement of DIC, because given two values from TA, DIC, p CO 2 and pH, the others can be derived [18] , [21] . At state 3′, the DIC (regardless of subscripts) and TA values are calculated using pH meas and assumed gas-solution equilibrium, i.e., CO 2 ( aq ) = 0.035 × p CO 2 , where 0.035 comes from Henry’s law constant of 35 mM bar −1 for CO 2 at room temperature. Because ΔTA 3′i→1 is known from Fig. 2c , TA 1 can be evaluated, and so can the TA values at other states. One way of obtaining DIC in all states except 3′ i and of obtaining ΔDIC values between all states is to use the known TA and CO 2 (aq), and we denote these values with subscript “TA–eq” (Table 1 ). This method is also used to construct the ideal cycles ( Supplementary Fig. 1 ). Another way to calculate DIC is to use the TA and pH meas without assuming gas-solution equilibrium. We denote DIC and ΔDIC calculated this way with subscript “TA−pH”. The ΔDIC between state 3′ i and 1 , i.e., 0.20 M, determined by flow meter and CO 2 sensor, i.e., ΔDIC flow,3′i→1 , is corroborated by ΔDIC TA−pH,3′i→1 , and ΔDIC TA−eq,3′i→1 (Table 1 ). Fig. 2: A CO 2 concentrating cycle with inlet pressure p 1 = 0.1 bar and exit pressure p 3 = 1 bar using a DSPZ-based flow cell at 40 mA cm −2 . Electrolytes comprised 10 mL 0.11 M DSPZ in 1 M KCl (negolyte, capacity limiting) and 35 mL 0.1 M K 4 Fe(CN) 6 and 0.04 M K 3 Fe(CN) 6 in 1 M KCl (posolyte, non-capacity limiting). a Current density. b Voltage. c Total alkalinity. d pH of the negolyte. States 3′ i , 1, 1′, 3 and 3′ f represent pH values before deacidification under 0.1 bar p CO 2 , after deacidification+absorption under 0.1 bar p CO 2 , after changing p CO 2 from 0.1 bar to 1 bar, after acidification+desorption under 1 bar and after changing p CO 2 from 1 bar to 0.1 bar, respectively. The detailed composition of these states is elaborated in Table 1 . e N 2 and CO 2 percentage in the upstream source gas, controlled by mass flow controllers. f Downstream CO 2 partial pressure. The baseline indicates p CO 2 = 0.1 bar. Inset: Zoomed-in view of downstream CO 2 partial pressure in between 0 < t < 2 h, where CO 2 capture takes place. g Downstream total gas flow rate; the baseline is 11.8 mL min −1 . Inset: Zoomed-in view of downstream gas flow rate (filtered) in between 0 < t < 2 h, where CO 2 capture takes place. Full size image Table 1 Summary of TA, p CO 2 , pH, DIC and ΔDIC. Full size table After CO 2 capture at 0.1 bar ( p 1 ) was completed, the headspace of the negolyte was switched to a pure CO 2 environment ( p 3 ) to prepare for CO 2 outgassing, i.e., going through process 1→1′ (Fig. 2e , t = 2.2 h). The drop in flow rate at t = 2.2 h and its return to the baseline at 2.5 h is caused by the combined effect of mismatched valve response rate in the MFCs (the N 2 MFC valve closes faster than the CO 2 MFC valve opens) and a small increase in DIC due to increased p CO 2 in the headspace. This increase in DIC, corresponding to ΔDIC 1→1′ , is difficult to quantify via the flowmeter and CO 2 sensor, but can be determined using pH meas (ΔDIC TA−pH,1→1′ ) or assuming gas-solution equilibrium (ΔDIC TA−eq,1→1′ ), which both give 0.03 M (Table 1 ). The acidification+CO 2 outgassing (process 1′→3) started at t = 3.2 h and ended at a little over 3.6 h (Fig. 2a–d, g ). Note that, unlike in process 3′ i →1, the CO 2 outgassing, which is observable from pH change and an increase in flow rate, (Fig. 2d, g ) lasted for no more than ten minutes after the acidification process (Fig. 2a, b ) finished. The outgassed CO 2 volume was 49 mL (Eq. 1 ), which is equivalent to ΔDIC flow,1′ →3 = −0.20 M. Once again, ΔDIC TA−pH and ΔDIC TA−eq agree with ΔDIC flow for the changes between states 1′ and 3. Starting from a little over t = 5.2 h, the headspace was filled with 0.1 bar CO 2 + 0.9 bar N 2 to recover the state 3’ for the next cycle (process 3→3′ f ). Like process 1→1′, there was a combined effect of valve response and additional CO 2 outgassing during process 3→3′ f , causing an increase in flow rate (Fig. 2g , t = 5.2 h to 5.6 h). Note that state 3′ f has slightly higher pH and 0.01 M more of TA and DIC than state 3′ i because of the influence of oxygen (Fig. 1c ). Calculation of ΔDIC flow,3→1 , molar cycle work, and productivity The discussion above shows how ΔDIC flow,3′i→1 and ΔDIC flow,1′→3 are obtained by gas flow measurement, but neither of these two quantities reflect the actual amount captured at 0.1 bar and released at 1.0 bar, because both states 3′ i and 1 are at p 1 = 0.1 bar while both states 1′ and 3 are at p 3 = 1 bar. The important quantity is the difference in DIC between states 3 and 1. With help of TA and pH measurements, ΔDIC flow,1→3 is evaluated as ΔDIC TA−pH,1→1′ + ΔDIC flow,1′ →3 = −0.17 M; equivalently, but with opposite sign, ΔDIC flow,3→1 = ΔDIC flow,3′ →1 + ΔDIC TA−pH, 3→3′ f = 0.17 M, i.e., 1.7 mmol CO 2 in a 10 mL negolyte volume. Because sufficient gas-solution equilibrium is approached (Fig. 2f, g ), ΔDIC TA−eq may also be used in place of ΔDIC TA−pH in such calculations, resulting in the same values of ΔDIC flow,1→3 and ΔDIC flow,3→1 . In this cycle, the deacidification work into the system, w deacidification , is 0.267 kJ and the acidification work, w acidification , is −0.119 kJ (Eq. 3 ). Dividing the cycle work, w cycle (Eq. 2 ), by 1.7 mmol CO 2 gives the molar cycle work of 87 kJ mol CO2 −1 . This value is already competitive with commercial amine scrubbing processes [4] , [6] , and it can be further decreased by using membranes with lower ohmic resistance or molecules with lower electron transfer overpotential [22] . The productivity measures the rate of a CO 2 separation process and may be evaluated by dividing ΔDIC flow,3→1 , i.e., 0.17 M, by the sum of the absorption time and the desorption time. The CO 2 absorption and desorption processes took 1.6 and 0.4 h, respectively, leading to a productivity of 0.085 M h −1 or 8.5 \(\times\) 10 −4 mol CO2 h −1 . The productivity should vary monotonically with current density because the desorption process is mostly limited by the rate of TA consumption, which is proportional to the rate of electrochemical oxidation. The solution-gas contacting area is quite limited in this experiment: gas was simply bubbled through the solution at a low rate (11.8 mL/min). Engineered contactor structures have many orders of magnitude higher contact area. Because the sorbent in this process is aqueous KOH, the contactor that is used for the concentrated alkaline process [9] might be adopted, for example, and a similar capture rate would be expected. Other factors such as solution concentration, gas flow rate, etc. also influence the productivity but analysis of such dependencies is beyond the scope of this study. Carbon capture cycles with p 1 = 0.1–0.5 bar at 40 mA cm −2 In order to understand how the electrical work depends on the inlet p CO 2 , we performed five cycles each at p 1 = 0.1 to 0.5 bar with p 3 = 1.0 bar (Fig. 3 ). The same cell components and negolyte as in Fig. 2 were used, and the posolyte was replaced with a fresh solution for each inlet condition to avoid oxygen-induced long-term cell imbalance (Fig. 1c ) [23] . 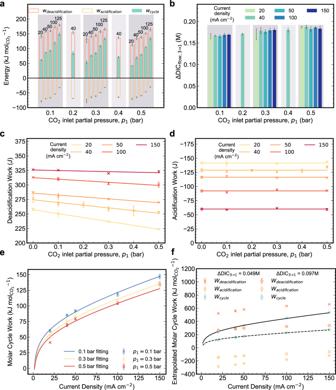Fig. 5: Summary of the experimental concentrating cycles performed under 20, 40, 50, 100 and 150 mA cm−2current densities andp1= 0.5, 0.4, 0.3, 0.2 and 0.1 bar. TA is total alkalinity and DIC is dissolved inorganic carbon. Electrolytes comprised 10 mL of 0.11 M DSPZ in 1 M KCl (negolyte) and 35 mL of 0.1 M K4Fe(CN)6and 0.04 M K3Fe(CN)6in 1 M KCl (posolyte). The error bars refer to standard deviation.aCO2molar deacidification, acidification, and cycle workvs. p1for current densities indicated above the bars, in mA cm−2. In both (a) and (b) the horizontal axis is categorical, and each shadowed region refers to a singlep1value.bΔDICflow,3→1vs p1for various current densities.cDeacidification workvs. p1for various current densities. The “x” markers refer to measured data. The deacidification work of the cycles under pure N2is used forp1= 0.0 bar.dAcidification work vs.p1for various current densities. The “x” markers refer to measured data. For each current density, the acidification work atp1= 0.0 bar (“o” markers) is chosen to be the average value of the work obtained at otherp1values at the same current density.eCO2molar deacidification, acidification and cycle work vs. current density forp1= 0.1, 0.3 and 0.5 bar. The curves are fitted using a Tafel model.fExtrapolated CO2molar deacidification, acidification and cycle work forp1= 0.4 mbar. Extrapolation is performed using deacidification and acidification work at 0.0 barp1in (c) and (d), and divided by ΔDICTA–eq,3→1atp1= 0.4 mbar obtained from Fig.4aandSupplementary Fig. 2b. The solid line refers to a Tafel model fit of CO2molar cycle work vs. current density assuming TA3’i= 0.11 M (ΔDIC3→1= 0.049 M) and the dashed line refers to the same fitting but assuming TA3′i= 0.0 M (ΔDIC3→1= 0.097 M). Supplementary Figure 5b shows that the CO 2 outgassing period is identical regardless of inlet p CO 2 because the exit p CO 2 is always 1 bar and the current density is always 40 mA cm −2 . In contrast, the capture period increases as inlet p CO 2 decreases ( Supplementary Fig. 5a ) because of the expected trend of reaction rate with decreasing reactant concentration. ΔDIC flow,3→1 values decrease as p 1 decreases (Fig. 4a ) because of greater ΔDIC during processes 1→1’ and 3→3’ (vertical arrows in Fig. 4c ) at smaller p 1 . The measured values closely align with the theoretical ΔDIC TA−eq,3→1 vs. p 1 curve (Fig. 4a ). Fig. 3: Twenty five CO 2 concentrating cycles with 0.5, 0.4, 0.3, 0.2, and 0.1 bar inlet pCO2 and 1 bar exit pCO2 at 40 mA cm −2 . Same cell and negolyte as in Fig. 2 were employed . a Current density. b Voltage. c pH of the negolyte. d N 2 and CO 2 percentage in the upstream source gas, controlled by mass flow controllers; total pressure 1.0 bar. e Downstream CO 2 partial pressure. f Downstream total gas flow rate. Full size image Fig. 4: Summary of the experimental concentrating cycles with different inlet p CO2 in Fig. 3 and the TA (total alkalinity)/pH/DIC (dissolved inorganic carbon) relations of the ideal cycles with corresponding experimental conditions. a ΔDIC flow extracted from Fig. 3e, f (colored “x” markers) and calculated ΔDIC TA−eq given TA 3′i = 0.11 M and ΔTA 3→1 = 0.21 M (lines). The black “x” marker refers to the result that ΔDIC for the ideal cycle equals 0.049 M when p CO 2 = 0.4 mbar. The error bars refer to the standard deviation. b pH vs . TA in the ideal cycles, assuming TA 3′ i = 0.11 M, ΔTA 3→1 = 0.21 M and gas-solution equilibrium. p 1 in the legends represents p CO 2 during the two-stage deacidification+CO 2 invasion process. The arrows indicate the direction of the processes in the experiments. c DIC vs . TA in the ideal cycles. d DIC vs . pH in the ideal cycles. Full size image This alignment permits us to estimate ΔDIC fow,3→1 for p 1 = 0.4 mbar and p 3 = 1 bar, i.e., similar to DAC conditions, by following the ΔDIC TA−eq,3→1 vs. p 1 curve to obtain a value of 0.049 M. Note that the ΔDIC TA−eq, 3→1 vs. p 1 curve shifts downward as TA 3’i increases ( Supplementary Fig. 3b ). This has relatively small impacts on ΔDIC TA−eq,3→1 with high p 1 , but it causes significant differences for small p 1 values. For example, when p 1 = 0.4 mbar, ΔDIC TA−eq,3→1 for TA 3′i = 0, 0.11 and 0.21 M is 0.097, 0.049 and 0.005 M, respectively ( Supplementary Figs. 1–3 ). Because ΔDIC 3→1 is in the denominator when CO 2 molar cycle work is calculated, lowering ΔDIC 3→1 increases the molar energy cost accordingly ( Supplementary Fig. 2b, c ). High TA 3’i should therefore be avoided, and a necessary step to achieve this goal is to limit the impact of oxidation of DSPZH 2 by oxygen (Fig. 1c ). Carbon capture cycles with p 1 = 0.1–0.5 bar at 20–150 mA cm −2 The average CO 2 molar cycle work under 40 mA cm −2 is compared with those obtained under 20–150 mA cm −2 (Fig. 5a and Supplementary Fig. 7 ). As current density increases at a fixed p 1 , the net cycle work increases as the required deacidification work increases and the acidification work returned decreases in magnitude; these trends are caused by increased ohmic, electron-transfer, and mass-transport overpotentials at higher current density [22] . It is noteworthy that we achieve 61.3 kJ mol CO2 −1 cycle work for p 1 = 0.1 bar and p 3 = 1 bar using a current density of 20 mA cm −2 , which is a competitive energy cost at a much higher current density compared to other electrochemical CO 2 separation methods for flue gas capture [24] , [25] . Fig. 5: Summary of the experimental concentrating cycles performed under 20, 40, 50, 100 and 150 mA cm −2 current densities and p 1 = 0.5, 0.4, 0.3, 0.2 and 0.1 bar. TA is total alkalinity and DIC is dissolved inorganic carbon. Electrolytes comprised 10 mL of 0.11 M DSPZ in 1 M KCl (negolyte) and 35 mL of 0.1 M K 4 Fe(CN) 6 and 0.04 M K 3 Fe(CN) 6 in 1 M KCl (posolyte). The error bars refer to standard deviation. a CO 2 molar deacidification, acidification, and cycle work vs. p 1 for current densities indicated above the bars, in mA cm −2 . In both ( a ) and ( b ) the horizontal axis is categorical, and each shadowed region refers to a single p 1 value. b ΔDIC flow,3→1 vs p 1 for various current densities. c Deacidification work vs. p 1 for various current densities. The “x” markers refer to measured data. The deacidification work of the cycles under pure N 2 is used for p 1 = 0.0 bar. d Acidification work vs. p 1 for various current densities. The “x” markers refer to measured data. For each current density, the acidification work at p 1 = 0.0 bar (“o” markers) is chosen to be the average value of the work obtained at other p 1 values at the same current density. e CO 2 molar deacidification, acidification and cycle work vs. current density for p 1 = 0.1, 0.3 and 0.5 bar. The curves are fitted using a Tafel model. f Extrapolated CO 2 molar deacidification, acidification and cycle work for p 1 = 0.4 mbar. Extrapolation is performed using deacidification and acidification work at 0.0 bar p 1 in ( c ) and ( d ), and divided by ΔDIC TA–eq,3→1 at p 1 = 0.4 mbar obtained from Fig. 4a and Supplementary Fig. 2b . The solid line refers to a Tafel model fit of CO 2 molar cycle work vs. current density assuming TA 3’i = 0.11 M (ΔDIC 3→1 = 0.049 M) and the dashed line refers to the same fitting but assuming TA 3′i = 0.0 M (ΔDIC 3→1 = 0.097 M). Full size image It is evident from Fig. 5b that ΔDIC flow,3→1 is independent of current density for a given value of p 1 . This occurs because varying current density changes only the rate of change in TA and not the value of ΔTA 3→1 , and sufficient reaction time was allowed to approach gas-solution equilibrium, whether the current density was low (Fig. 2f, g ) or high ( Supplementary Fig. 9 ). The consistent ΔTA 3→1 across various current densities is supported by the consistent charge/discharge capacities ( Supplementary Fig. 8 ). The slight variations in ΔTA and ΔDIC were caused by occasional foaming or negolyte droplets clinging to the wall of the reservoir, both of which cause small amounts of charge capacity to be instantaneously inaccessible from time to time. In contrast, increasing p CO 2 at the inlet raises ΔDIC flow,3→1 (Fig. 5b ), for the reason explained in the discussion of Fig. 4d . In addition to the cycle results presented in Fig. 5 , five cycles with p 1 = 0.05 bar and p 3 = 1 bar and current density being 40 mA cm −2 were tested under faster negolyte pumping to enhance mass transport rates, yielding an average cycle work of 92.6 kJ mol CO2 −1 ( Supplementary Fig. 10 ). Estimate of molar cycle work at p 1 = 0.4 mbar and p 3 = 1 bar Because of the limited sensitivity of our equipment, a direct measurement of CO 2 molar cycle work at p 1 = 400 ppm and p 3 = 1 bar, i.e., similar to DAC conditions, is currently infeasible in our laboratory, but we can extrapolate the molar cycle work under these conditions using the results obtained from p 1 = 0.1–0.5 bar. However, a simple linear regression of the molar cycle work from higher p 1 values to p 1 = 0.4 mbar does not guarantee accurate extrapolation because the deacidification work (Fig. 5c ), i.e., part of the numerator in the calculation of molar cycle work (Eqs. ( 2 )–( 4 ) in the “Methods” section), scales linearly with p 1 , whereas ΔDIC flow,3→1 , i.e., part of the denominator in the calculation of molar cycle work (Eq. ( 4 ) in the method section), scales non-linearly with p 1 (Fig. 4a, d and Supplementary Fig. 3b ). Therefore, we evaluate the molar cycle work at p 1 = 0.4 mbar by separately calculating ΔDIC flow,3→1 and the cycle work (i.e., the sum of the experimental deacidification work (Fig. 5c ) and the acidification work (Fig. 5d )). The deacidification work at p 1 = 0.4 mbar is simply approximated by the deacidification work under a pure N 2 atmosphere, i.e., 0.0 bar p CO 2 (Fig. 5c ); the reason that deacidification work decreases with increasing p 1 is that increasing p 1 lowers the average negolyte pH, which in turn decreases the cell voltage and thereby decreases the work (Eq. 3 in the “Methods” section). The acidification work is always the same regardless of p 1 because p 3 is always 1 bar and ΔTA 3→1 is always the same (hence the flat lines in Fig. 5d ); therefore, for p 1 = 0.0 bar we use the average acidification work from higher p 1 values. As for ΔDIC flow,3→1 at p 1 = 0.4 mbar, we assume it is equal to the value of ΔDIC TA–eq,3→1 in the ideal cycle at the same pressure. We have shown that measured (ΔDIC flow,3→1 ) and ideal cycle (ΔDIC TA–eq,3→1 ) values of ΔDIC 3→1 at p 1 = 0.1–0.5 bar agree very well (Fig. 4a , blue curve). With TA 3’i = 0.11 M and ΔTA 3→1 = 0.21 M, the ideal cycle value of ΔDIC TA–eq,3→1 at p 1 = 0.4 mbar and p 3 = 1 bar is 0.049 M (Fig. 4a , Supplementary Fig. 2b ). The molar cycle work for various current densities, evaluated by dividing the sum of deacidification and acidification work at p 1 = 0.0 bar by ΔDIC TA–eq,3→1 of 0.049 M, is shown in Fig. 5f . Figure 5f suggests that the molar cycle work at 20 mA cm −2 is 237.4 kJ mol CO2 −1 . This is on par with the concentrated KOH process [9] . However, if there is no initial alkalinity, i.e., TA 3’i = 0.0 M, and the same ΔTA 3→1 = 0.21 M is kept, the cycle work may be cut in half to 121.0 kJ mol CO2 −1 ; this occurs because of the nearly doubled ΔDIC flow,3→1 of 0.097 M despite similar cycle work ( Supplementary Figs. 2 and 3 ). The non-linear molar cycle work trend was fitted with a Tafel model, which suggests 72.8 and 98.1 kJ mol CO2 −1 at 5 and 10 mA cm −2 , respectively (ESI, Non-Linear Fit of Molar Cycle Work With Tafel Model). In addition, due to its solubility of 0.7 M in aqueous solution [18] , DSPZ can induce a ΔTA 3→1 or Δ[OH − ] of 1.4 M and thereby potentially yield even lower molar cycle work ( Supplementary Fig. 4 ) Comparison with existing technologies Table 2 summarizes some of the emerging technologies for point source capture, DAC, and direct ocean capture (DOC), where CO 2 is removed from seawater, allowing more CO 2 uptake by the ocean. Many approaches to DAC have used aqueous alkaline solutions [2] , [9] or solid amine-based adsorption methods [2] , [24] , which require thermal excursions to release captured CO 2 . One of the state-of-the-art DAC approaches relies on concentrated (2–5 Molar) alkaline solutions on a high-area contactor to absorb CO 2 and transform it into aqueous K 2 CO 3 and KHCO 3 . These are then converted into solid CaCO 3 in a pellet reactor by mixing the aqueous carbonates with Ca(OH) 2 . Releasing the CO 2 requires heating the CaCO 3 to 900 °C in an oxygen-fired calciner, which costs 264–296 kJ/molCO 2 [2] , [9] . Another, less mature, aqueous approach uses amino acids for the carbon capture step and undergoes a subsequent sorbent regeneration cycle employing solid bis-iminoguanidine carbonate precipitation and CO 2 release through heating to >100 °C; this cycle requires 152–422 kJ/molCO 2 , depending on the type of guanidine, because a significant portion of the energy contributes to removing the undesirable hydrate from guanidine carbonate crystal [10] , [16] . Solid sorbent DAC, mostly based on solid amine absorption and release through thermal and/or pressure swing, allows reduced heating requirements (~100 °C), but amine decomposition may lead to high operational and end-of-life costs [2] , [26] , [27] , [28] . Table 2 Comparison of this work and emerging technologies for DAC, DOC, and point source capture. CO 2 separation work with “th” subscript denotes thermal energy inputs, whereas “e” subscript denotes electrical work input. Full size table Electrochemical carbon capture methods may offer solutions to overcome the high sorbent regeneration energy penalty and sorbent decomposition issues. Electrochemically mediated point source carbon capture methods [7] , [24] , [29] , at low current densities, have exhibited lower energetic costs than amine-scrubbing methods. In addition, CO 2 removal from ocean water, which restores the CO 2 capture capability of oceans, via electrochemical methods such as bipolar membrane electrodialysis (BPMED), have shown promisingly low energetic cost [12] , [13] . However, the demonstrated works exhibited either low current density (slow kinetics) or low voltage efficiency. In addition, the high water-handling requirement of direct ocean capture adds significantly to the energetic cost. The performance of our pH-swing flow cell, demonstrated for capture at 0.1 bar and projected for 0.4 mbar appears competitive compared with existing technologies, not only in terms of energetic cost with cheap electricity from renewable sources, but also because of much larger applicable current density (Table 2 ) [30] . Additionally, the all-liquid configuration obviates the need for the precipitation and heating of solid carbonates. Furthermore, the compatibility with an aqueous electrolyte of non-volatile, non-corrosive and potentially low-cost organic molecules implies that a carbon capture technology based on this concept has the potential for wide scale practical implementation. Electrochemical rebalancing It is clearly difficult to avoid O 2 in either DAC or flue gas capture because the source gas contains 20% and 3−5% O 2 , respectively. In the short term, the oxidation of DSPZH 2 by O 2 incurs an instantaneous loss in Coulombic efficiency. In the long term the cell will go out of balance, accumulating oxidized species in both electrolytes and TA 3’i , KOH, and DIC 3’i in the negolyte (Fig. 1c ) [23] . As a result, ΔDIC 3→1 will shrink without a concomitant decrease in cycle work ( Supplementary Fig. 2b ), leading to an increase in CO 2 molar cycle work ( Supplementary Fig. 2c ). Eventually, the cell will no longer operate because both electrolytes are completely oxidized. As shown in Fig. 6a, b , as soon as the headspace was opened to air the Coulombic efficiency decreased to ~65%, and by the 20th subsequent cycle the cell lost all capacity due to depletion of reduced species, i.e., [K + ] 4 [Fe II (CN) 6 ] 4− , in the posolyte side. The negolyte pH also increased from near neutral to almost 14 during air exposure ( Supplementary Fig. 14b ). Development of oxygen-insensitive molecules may alleviate the problem caused by oxygen, but even if a tiny amount of Coulombic efficiency loss, e.g., 0.1%, took place every cycle, the effect is cumulative and will eventually lead to an out-of-balance cell problem (Fig. 1c ). Fig. 6: The capacity fade caused by O 2 on Fe(CN)6|DSPZ cell cycling (a–c) and its mitigation by the electrochemical rebalancing method (d–f). a Charge capacity vs. cycle number of the cell under pure N 2 atmosphere. The first cycle has much higher deacidification capacity due to residual oxygen. b Charge capacity vs. cycle number of the same cell from ( a ) under air. Capacity fades quickly because of the depletion of K 4 Fe(CN) 6 in the posolyte. c Charge capacity vs . cycle number of the cell from ( b ) under pure N 2 atmosphere, after the electrochemical rebalancing step. The first cycle has much higher deacidification capacity due to residual oxygen. d Current density, ( e ) voltage, ( f ) posolyte and negolyte pH during the electrochemical rebalancing step. Full size image Here we demonstrate the efficacy of the electrochemical rebalancing method. The method successfully recovers the pH of the negolyte and the capacity of the cell, which is thrown out-of-balance by O 2 -induced side reactions. The electrochemical rebalancing process comprises the cathodic reaction [K + ] 3 [Fe III (CN) 6 ] 3− + e − → [K + ] 4 [Fe II (CN) 6 ] 4− in the posolyte and the anodic oxygen evolution reaction, OH − → 2 e − + ½O 2 , in the negolyte. 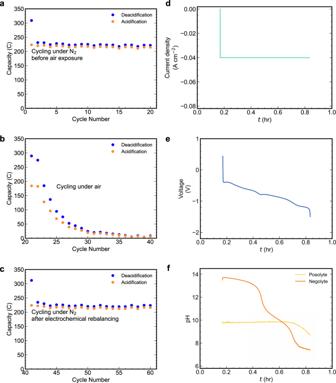Fig. 6: The capacity fade caused by O2on Fe(CN)6|DSPZ cell cycling (a–c) and its mitigation by the electrochemical rebalancing method (d–f). aCharge capacity vs. cycle number of the cell under pure N2atmosphere. The first cycle has much higher deacidification capacity due to residual oxygen.bCharge capacity vs. cycle number of the same cell from (a) under air. Capacity fades quickly because of the depletion of K4Fe(CN)6in the posolyte.cCharge capacityvs. cycle number of the cell from (b) under pure N2atmosphere, after the electrochemical rebalancing step. The first cycle has much higher deacidification capacity due to residual oxygen.dCurrent density, (e) voltage, (f) posolyte and negolyte pH during the electrochemical rebalancing step. Figure 6d–f shows the cell behavior when the electrochemical rebalancing process is applied to the completely out-of-balance cell (Fig. 6b ). The process starts when a constant current of −40 mA cm −2 is applied (Fig. 6d ). The voltage immediately drops from 0.2 V to negative values because both the cathodic and anodic half reactions are at ~0.4 V vs. SHE at pH 14, and there is high activation overpotential for the oxygen evolution reaction (Fig. 6e ). As the rebalancing process progresses, the pH of the negolyte side decreases (Fig. 6f ), causing the anodic half reaction to shift to higher potential, thereby further decreasing the cell potential (Fig. 6e ). The sharp drop in voltage to a plateau near 0.8 h indicates the completion of the electrochemical rebalancing process. Figure 6c shows the post-rebalancing cell capacity, which is almost identical to that prior to air exposure (Fig. 6a ), indicating that essentially all lost capacity due to imbalance has been restored. The capacity accounting for all the electrons passed in the electrochemical rebalancing step is 476.8 C, which is within 1% of the theoretical capacity (473 C) of the posolyte side, suggesting a complete recovery of the K 4 Fe(CN) 6 and minimal side reactions other than oxygen evolution. The posolyte pH did not change much during the process because the cathodic half-reaction is not proton-coupled (Fig. 6f ). The neutral pH of the negolyte at the end of the process indicates that virtually all of the accumulated hydroxide has been removed (Fig. 6f ). The undiminished capacity also suggests that this method is not detrimental to DSPZ. Supplementary Figure 14 shows that the electrolytes, after electrochemical rebalancing, have the same carbon-capture capability as the original electrolytes, and the NMR spectra in Supplementary Fig. 15 suggest no new species was generated during the process. Hence, the electrochemical rebalancing process is a very effective method to remove the adverse effect of oxygen in DSPZ-based carbon capture flow cells. This method has potentially broad application beyond DSPZ and carbon capture, e.g., mitigating the oxygen effect in flow batteries with air or pH-sensitive electrolytes (ESI, More on Electrochemical Rebalancing) [23] , [34] , [35] , [36] , [37] , [38] , [39] , [40] , [41] . The overall energy cost is 378 J, which is approximately 1.4 times of the cost of one deacidification half cycle at 40 mA cm −2 (Fig. 5c ). This will be a significant cost if the electrochemical rebalancing is applied every few cycles, which may be necessary for a DSPZ-based system for DAC, but if the negolyte molecule is much less air sensitive or the source gas has lower oxygen content, requiring electrochemical rebalancing less frequently than once every few tens of carbon capture/release cycles, the cost will be negligible. The development of oxygen-insensitive molecules for this purpose is the subject of active research. In this work, we have performed a series of CO 2 concentrating cycles using a DSPZ-based flow cell with electrochemically induced pH swings, and the cycle work under different inlet partial pressures and current densities was analyzed and compared. We demonstrated a 61.3 kJ mol CO2 −1 cycle work for CO 2 separation for capture at p 1 = 0.1 bar and release at p 3 = 1 bar, at a current density of 20 mA cm −2 . If TA 3′i is carefully maintained at a low level, the extrapolated separation work for p 1 = 0.4 mbar and p 3 = 1 bar is 121 kJ mol CO2 −1 at 20 mA cm −2 and this figure can be further lowered if a higher concentration of DSPZ or another PCET-active molecule is used. Our Tafel model suggests that molar cycle work at p 1 = 0.4 mbar may be even lower than 100 kJ mol CO2 −1 at smaller current densities . Recognizing the inevitable O 2 -induced imbalance and capacity fade in both point source capture and DAC, we report an electrochemical rebalancing method that recovers the initially healthy cell composition. This method can serve as a convenient tool for mitigating oxygen-related problems in many electrochemical applications. We anticipate that the low energetic cost of the pH swing cycles and the effectiveness of the oxygen mitigation method demonstrated here will accelerate the techno-economic competitiveness of electrochemically-driven carbon capture systems. Materials and characterization All chemicals were purchased from Sigma-Aldrich or Acros Organics and were used as received. The synthetic method for DSPZ is adapted from previous work [18] . In this work, sodium hydride was used to deprotonate the reaction intermediate phenazine-2,3-diol (DHPZ) instead of sodium methoxide ( Supplementary Fig. 17 ). Flow cell experiments Flow cell experiments were constructed with cell hardware from Fuel Cell Tech. (Albuquerque, NM), assembled into a zero-gap flow cell configuration, similar to a previous report [18] . Pyrosealed POCO graphite flow plates with serpentine flow patterns were used for both electrodes. Each electrode comprised a 5 cm 2 geometric surface area covered by a stack of four sheets of Sigracet SGL 39AA porous carbon paper pre-baked in air for 24 h at 400 °C. The outer portion of the space between the electrodes was gasketed by Viton sheets with the area over the electrodes cut out. Torque applied during cell assembly was 80 lb-in on each of eight 1/4-28 bolts. The membrane used is a Fumasep E620(K) CEM. Cell electrolytes comprised 10 mL 0.11 M DSPZ in 1 M KCl (negolyte, capacity limiting, theoretical capacity 212 C) and 35 mL 0.1 M K 4 Fe(CN) 6 and 0.04 M K 3 Fe(CN) 6 in 1 M KCl (posolyte, non-capacity limiting, theoretical capacity 473 C). For every new CO 2 capture cycle condition (changing current density or inlet p CO 2 ), the posolyte was replaced with a fresh solution and the negolyte was acidified by adding drops of 1 M HCl to remove the accumulating effect of oxygen side reactions. 10 μL of antifoam B emulsion purchased from Sigma-Aldrich was added into the negolyte solution before cell cycling to suppress foam formation. Posolytes were fed into the cell through fluorinated ethylene propylene (FEP) tubing at a rate of 100 mL min −1 controlled by a Cole-Parmer 6 Masterflex L/S peristaltic pump, and the negolytes were circulated at the same rate controlled by a Cole-Parmer Masterflex digital benchtop gear pump system. Both posolyte and negolyte upstream gas was controlled by Sierra Smart Trak 50 Mass Flow Controllers. The flowmeter used in the downstream of negolyte headspace was a Servoflo FS4001-100-V-A. The CO 2 sensor was an ExplorIR-W 100% CO 2 sensor purchased from co2meter.com. A Mettler Toledo pH electrode LE422 was used to monitor electrolyte pH. As shown in Fig. 1b , a drierite drying tube (Cole Parmer) was placed in between the sensors and the negolyte chamber to reduce the humidity level of the gas. Glassy carbon (BASi MF-2012, 3.0 mm diameter) was used as the working electrode for all three-electrode CV tests. A Ag/AgCl reference electrode (BASi MF-2052, pre-soaked in 3 m NaCl solution), and a graphite counter electrode were used for CV tests. CV tests and cell cycling were performed using a Gamry Reference 3000 potentiostat. All cycles were galvanostatic until the 1.65 and 0.2 V voltage cutoff for deacidification and acidification, respectively, were reached, and then went through a potentiostatic process until the current reached 10 mA cm −2 . In the CO 2 cycles with p 1 = 0.1, 0.2, 0.3, 0.4, and 0.5 bar, the MFCs set the initial negolyte headspace atmosphere to be p 1 , which was then switched back and forth between p 1 and p 3 every three hours. In the cycles with p 1 = 0.05 bar, the switching period was 5 h. Calculation of absorbed or released CO 2 amount Because the deviation from baseline in Fig. 2g is solely caused by CO 2 absorption, the amount of CO 2 captured is calculated by integrating over the difference between the recorded flow rate and the baseline in between 0.2 and 1.8 h, i.e., 
    Q_CO_2=∑_n=t_i^t_f(V̇^base-V̇^n)Δ t
 (1) where \({Q}_{{{{{{\rm{C{O}}}}}}}_{2}}\) is the volume of CO 2 , t i is the start time, t f is the final time, V̇ n is the instantaneous volumetric flow rate at n th data recording time t n , V̇ base is the baseline flow rate of 11.6 mL min −1 , and Δ t is the time difference between successive measurements. Calculation of deacidification, acidification, and cycle work The net cycle work is calculated by combining the work required for deacidification in process 3′ i →1 and the work returned by acidification in process 1′→3, i.e., 
    w_cycle=w_deacidification+w_acidification
 (2) The work in a process is calculated by summing over the product of voltage (Fig. 2a ) and current (Fig. 2b ), i.e., 
    w_deacidification/acidification=∑_n=t_i^t_fV^nj^nAΔ t
 (3) where V n is the cell voltage at the n th data recording time t n , j n is the current density at t n and A is the active geometric area of 5 cm 2 . The molar cycle work \(\bar{w}\) is calculated by dividing w cycle by −ΔDIC flow,1→3 or ΔDIC flow,3→1 : 
    w̅=w_cycle/DIC_flow,3→ 1
 (4) where ΔDIC flow,1→3 = ΔDIC TA−pH,1→1′ + ΔDIC flow,1′ →3 and ΔDIC flow,3→1 = ΔDIC flow,3′ →1 + ΔDIC TA−pH, 3→3′ f . For high current densities (100 and 150 mA cm −2 ), we use ΔDIC TA−eq,1→1′ and ΔDIC TA−eq, 3→3′ f instead of ΔDIC TA−pH,1→1′ and ΔDIC TA−pH, 3→3′ f , respectively, because of an artifact in the pH measurement at high current density, tentatively attributed to crosstalk between potentionstat lines. We explain in the main text that ΔDIC TA−pH and ΔDIC TA−eq are interchangeable when the pH measurement is valid.